Functional links between stability and reactivity of strontium ruthenate single crystals during oxygen evolution In developing cost-effective complex oxide materials for the oxygen evolution reaction, it is critical to establish the missing links between structure and function at the atomic level. The fundamental and practical implications of the relationship on any oxide surface are prerequisite to the design of new stable and active materials. Here we report an intimate relationship between the stability and reactivity of oxide catalysts in exploring the reaction on strontium ruthenate single-crystal thin films in alkaline environments. We determine that for strontium ruthenate films with the same conductance, the degree of stability, decreasing in the order (001)>(110)>(111), is inversely proportional to the activity. Both stability and reactivity are governed by the potential-induced transformation of stable Ru 4+ to unstable Ru n>4+ . This ordered(Ru 4+ )-to-disordered(Ru n>4+ ) transition and the development of active sites for the reaction are determined by a synergy between electronic and morphological effects. Functional oxides have a significant role in a number of technologically important areas, including superconductivity, magnetism and heterogeneous catalysis [1] , as well as in electrochemical technologies and processes that use both aqueous electrolytes [2] , [3] and organic solvents [4] , [5] , [6] . One class of electrochemical reactions of particular significance is the oxygen electrochemistry on metal oxide materials [7] , [8] , [9] , specifically the production (evolution) of oxygen in electrolysers, metal–air batteries and electrometallurgy [7] . Most conventional commercial electrolysers use alkaline electrolytes and operate at relatively modest current densities with cell voltages of ~1.8–2.0 V (refs 7 , 10 ). The cathodic half-cell reaction in alkaline electrolytes is the hydrogen evolution reaction (2H 2 O+2e − =H 2 +2OH − ) in which hydrogen and hydroxyls are produced from the water splitting reaction [11] , [12] . The hydroxyl ions that are generated at the cathode are consumed at the anode where the more complex oxygen evolution reaction (OER; 4OH − =O 2 +2H 2 O+4e − ) takes place at overpotentials (defined as the difference between the thermodynamic potential for the water splitting reaction, 1.229 V, and the operating potentials) higher than 0.5 V (refs 13 , 14 ). The chief goal in the development of practical anode electrocatalysts is to find electronically conductive and stable oxides with activity at low overpotentials—all three demanding requirements that have severely hampered the use of oxide materials in electrochemical systems. So far, a wide variety of anode materials have been evaluated (tested) for the OER in alkaline environments, ranging from noble metal oxides (for example, RuO 2 and IrO 2 ) to various combinations of the rutile-type (for example, NiO 2 , MnO 2 , PbO 2 and TiO 2 ) (refs 15 , 16 ) and spinel-type (for example, Co 3 O 4 and Fe 3 O 4 ) oxide materials [17] , [18] , as well as the more complex pyrochlore phases (for example, A 2 B 2 O 7 , where A=Pb and Bi; and B=Ru and Ir) and perovskite-type (for example, ABO 3 , where A=Ca, Sr, La, Na and so on; and B=Ti, Ru, Ni, Co and so on) oxide structures [19] , [20] , [21] , [22] . In basic environments with high pH values, the most active anode oxide is RuO 2 , which is highly conductive but very expensive and unstable [2] , [22] , thus leading to a huge practical consequence—high cost of catalyst and short lifetime of operation. In an effort to reduce the high cost associated with use of noble oxide catalysts, the focus has very recently shifted towards spinel- and perovskite-type structures which, as in the past [21] , [23] , have shown some promising activity for the OER in alkaline solutions. The selection of such cost-effective oxide materials, however, was pursued chiefly by testing the activity of high-surface area powders (in the micron size range) or thin polycrystalline films [24] . Two important advantages of using high-surface area oxide powders supported on a conductive support are that the conductivity issue can be overcome, as well as that the synthesis methods are well established [25] , [26] , [27] , [28] . As for many other electrochemical reactions [29] , however, the use of such high-surface area oxide materials poses many key fundamental limitations, including (i) the lack of reliable procedures for determining the specific surface area of oxide materials; (ii) the absence of functional links between the nature of the active sites and their stability during the OER; and (iii) the inability to develop structure–function relationships between the electrochemical reactivity and the atomic-level surface structure. Given that the established structure–function relationships on metal surfaces ultimately formed the basis for a predictive ability in tailor-making commercial catalysts [30] , [31] , [32] , [33] , [34] , study of the OER on atomically smooth complex oxide surfaces is a topic of broad scientific significance as well as enormous technological importance. Here, we demonstrate that it is indeed possible to develop a distinctive experimental strategy that will enable the elucidation of structure–function relationships for the OER on well-characterized strontium ruthenate (SrRuO 3 ) single-crystal thin films (denoted hereafter as SRO(hkl)) prepared on Nb-doped SrTiO 3 (STO(hkl)) single-crystal substrates. To study the effect of conductance, we develop a unique methodology for modifying the ohmic resistance arising from the substrate–film structure as well as the Schottky barriers that form at the SRO–STO interface. We find that the degree of stability of the SRO surfaces [(001)>(110)>(111)] is inversely proportional to the OER activity. In addition, both stability and reactivity are controlled by the potential-induced transformation of stable Ru 4+ to unstable Ru n>4+ , resulting in the electrochemical corrosion of Ru followed by the chemical corrosion of Sr atoms. This structure-sensitive ‘ordered(Ru 4+ )-to-disordered(Ru n>4+ )’ transition and the development of ‘active sites’ for the OER is determined by a synergy between electronic effects (surface energy) and morphological effects (surface defects). On the bases of these results, we propose that the activity is controlled by the surface density of defects (for example, stability of Ru cations) rather than the binding energy between the substrate and oxygenated species. We conclude that the OER on SRO(hkl) films must be based on a careful equilibrium between two opposing effects—the balance between active but unstable Ru n>4+ sites with stable and inactive Ru 4+ sites. Structural and electrochemical characterizations We begin by presenting the in situ X-ray scattering data used to determine the morphology of as-grown SRO(hkl) films at 0.95 V, a potential where the structure and physical properties of as-grown SRO(hkl) films were found to be stable. From the specular rod scans (that is, scans along the direction normal to the film surface) shown in Fig. 1a–c , three distinguishing features (labelled as S, F and Kiessig fringes (KF)) are noteworthy. The appearance of sharp substrate peaks (S) confirms that the supports are well-ordered single crystals with (001), (110) or (111) orientation [35] . The measured locations of the SRO(hkl) film peaks (denoted as F) provide a means of determining the precise vertical lattice spacing of the films. From these scans, as well as those performed on non-specular rods [36] , we find the following: (i) the SRO(hkl) films are high-quality single crystals that are epitaxially oriented and lattice-matched with the substrate (that is, the films are laterally compressed by ~0.64% (ref. 37 ) to match the smaller lattice parameter of STO(hkl); and (ii) the films exhibit an out-of-plane expansion of the lattice parameter relative to the bulk lattice parameter of SRO as a consequence of this lateral strain (that is, the film peaks are found at smaller reciprocal lattice vector ( Q ) than would be expected for bulk SRO). Note that the increase of the free energy induced by the lateral strain is smaller than 15 meV per unit cell [38] and is expected to have only a minor effect on the surface activities under discussion [39] . The atomic configurations and lattice spacings of the three different orientations of SRO(hkl) films investigated in this study are indicated in Fig. 1d–f . 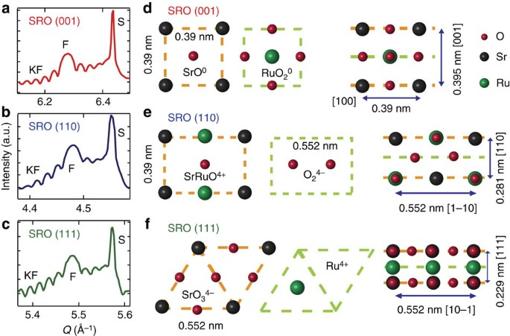Figure 1: Crystal structures of SrRuO3(SRO) (hkl) thin films. (a–c) SRO(001), (110) and (111) are denoted by SRO films grown on Nb-doped SrTiO3(STO)(001), (110) and (111) substrates, respectively, in the pseudocubic notation. Specular rod scans of (a) SRO(001), (b) SRO(110) and (c) SRO(111) films at a 0.95 V in 0.1 M KOH. Peaks S, F and KF represent the STO Substrate Bragg peak, the SRO Film Bragg peak and Kiessig Fringes, respectively. (d–f) Schematic representations of possible in-plane termination layers (orange and green dashed line) and stacking for three different orientated model systems: (d) SRO(001), (e) SRO(110) and (f) SRO(111). SRO(001) has non-polar layers, for example, RuO20and SrO0, whereas SRO (110) and SRO (111) possess polar layers (+4 and −4). Figure 1: Crystal structures of SrRuO 3 (SRO) (hkl) thin films. ( a – c ) SRO(001), (110) and (111) are denoted by SRO films grown on Nb-doped SrTiO 3 (STO)(001), (110) and (111) substrates, respectively, in the pseudocubic notation. Specular rod scans of ( a ) SRO(001), ( b ) SRO(110) and ( c ) SRO(111) films at a 0.95 V in 0.1 M KOH. Peaks S, F and KF represent the STO Substrate Bragg peak, the SRO Film Bragg peak and Kiessig Fringes, respectively. ( d – f ) Schematic representations of possible in-plane termination layers (orange and green dashed line) and stacking for three different orientated model systems: ( d ) SRO(001), ( e ) SRO(110) and ( f ) SRO(111). SRO(001) has non-polar layers, for example, RuO 2 0 and SrO 0 , whereas SRO (110) and SRO (111) possess polar layers (+4 and −4). Full size image Information about the film thickness and surface roughness is assessed by analysing the so-called KF [40] (also labelled as KF in Fig. 1a–c ) that arise from the interference between the X-rays scattered from the top and bottom interfaces of the film. The appearance of periodic KF on both sides of the Bragg peak for SRO(hkl) films is a clear indication that at 0.95 V, the films are smooth. In addition, from the scans shown in Fig. 1a–c , we determine that all three as-grown films have thicknesses in the range 20–30 nm and an average RMS roughness less than 1 nm (2 unit cells). The surface quality of all three as-grown SRO thin films was further studied by ex situ atomic force microscopy (AFM), which shows roughness values that depend slightly on the surface orientation. Although the AFM image of SRO(001) ( Fig. 2a (inset)) reveals that the surface is smooth and atomically flat, the AFM image of SRO(111) is consistent with a surface having a higher density of defects. This is not surprising considering that of all possible orientations, the epitaxial growth of SRO(001) is known to provide the best film quality. Nevertheless, from the X-ray scattering and AFM data, we conclude that high-quality SRO(hkl) films were grown, and that they remained essentially unchanged in alkaline environments between +0.05 and +0.95 V ( Supplementary Figs 1 and 2 ). For a reaction that occurs above 0.95 V, however, to establish correlations between reactivity and the atomic-level surface structure, it is of paramount importance to determine first the conductance and then the stability for each of the three orientations of oxide films. 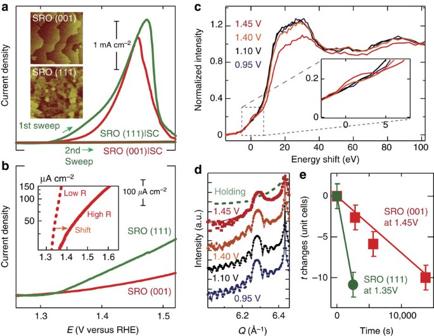Figure 2: Operando X-ray scattering and spectroscopy studies of SRO films. (a) Current density measured (1st and 2nd sweep) at certain potentials of SRO(001) and SRO(111) side-connected with conducting paths from the top surface to the bottom substrate, denoted by SRO|SC. The insets show atomic force microscopy (AFM) topography of SRO(001) (3 × 3 μm2) and (111) (0.5 × 0.5 μm2) pristine films. Both roughness root-mean-square (r.m.s.) values are below 0.5 nm. (b) Current density measured at certain potentials of SRO(001) and SRO(111) without the side connection denoted by SRO. The inset is the comparison between SRO(001)|SC and SRO(001). (c) Ru K-edge X-ray absorption spectra of SRO (001) film as a function of applied potential indicate a valence shift when the potential was increased from 1.40 to 1.45 V. The inset enlarges the pre-edge of the normalized absorption values at the potentials I—IV (I=0.95, II=1.10, III=1.40 and IV=1.45 V). (d) Specular rod scans of SRO(001) film at four potentials and extended hold at 1.45 V. Symbols and solid lines represent the experimental data and the fitting curves, respectively. (e) Dissolution rates (tchanges=t−ti, wheretiis the initial thickness at a given potential) of SRO(001) (red square) and SRO(111) (green circle) are 2.5 and 15.6 unit cells h−1, measured at 1.45 and 1.35 V, respectively. Figure 2: Operando X-ray scattering and spectroscopy studies of SRO films. ( a ) Current density measured (1st and 2nd sweep) at certain potentials of SRO(001) and SRO(111) side-connected with conducting paths from the top surface to the bottom substrate, denoted by SRO|SC. The insets show atomic force microscopy (AFM) topography of SRO(001) (3 × 3 μm 2 ) and (111) (0.5 × 0.5 μm 2 ) pristine films. Both roughness root-mean-square (r.m.s.) values are below 0.5 nm. ( b ) Current density measured at certain potentials of SRO(001) and SRO(111) without the side connection denoted by SRO. The inset is the comparison between SRO(001)|SC and SRO(001). ( c ) Ru K-edge X-ray absorption spectra of SRO (001) film as a function of applied potential indicate a valence shift when the potential was increased from 1.40 to 1.45 V. The inset enlarges the pre-edge of the normalized absorption values at the potentials I—IV (I=0.95, II=1.10, III=1.40 and IV=1.45 V). ( d ) Specular rod scans of SRO(001) film at four potentials and extended hold at 1.45 V. Symbols and solid lines represent the experimental data and the fitting curves, respectively. ( e ) Dissolution rates ( t changes= t − t i , where t i is the initial thickness at a given potential) of SRO(001) (red square) and SRO(111) (green circle) are 2.5 and 15.6 unit cells h −1 , measured at 1.45 and 1.35 V, respectively. Full size image As already mentioned, the inherently low electronic conductivity of oxide materials is one of three key problems that have hampered the resolution of many fundamental issues related to oxide electrochemistry. In general, while high electronic conductivity provides an opportunity to focus exclusively on the synergetic structure–function relationships between the activity and stability of oxides for highly unstable materials such as SRO ( vide infra ) the very same properties can limit the possibility of monitoring in situ the potential-dependent variations in morphology and electronic properties of the films. To learn more about possible conductivity effects, however, we prepared two types of STO/SRO sample geometries, both with the same film structure but with different resistances at the junction between the SRO film and the STO ranging from 100 Ω for high-conductance samples (SRO(hkl)|SC (side connection)) to >1 kΩ for low-conductance samples (SRO(hkl)). The resistance is controlled by the Schottky barrier created at the STO–SRO interface. More details on the electrodes can be found in the Methods section. In situ X-ray studies As an illustration, Fig. 2a shows typical current–potential curves (the so-called polarization curves) for the OER of highly conductive SRO(111) and SRO(100) films. Interestingly, both polarization curves show an unusual shape: while the current density initially increases with potential, as expected, it abruptly decreases at high overpotentials showing deactivation. Such current–potential behaviour is typical for electrochemical reactions in which the rate of reaction is determined by decreasing the number of active sites either via the adsorption of spectator species or dissolution of active centres [41] , [42] ; however, such behaviour has never been observed for the OER, at least when using bulk electrodes and high-surface area nanoparticles. As we will provide more evidence in the subsequent sections, we show below that these unusual shapes of polarization curves arise from a continuous degradation of the SRO(hkl) films during the OER, leading to a complete loss of the active Ru sites required for efficient transformation of the hydroxyl ions to O 2 and H 2 O. A closer inspection of Fig. 2a shows that the OER is a structure-sensitive reaction, that is, the SRO(111) film is more active than the SRO(001) film—an observation that, to the best of our knowledge, has never been reported for any single-crystal oxide material. As may be expected, the low-conductance SRO samples exhibit slower OER kinetics, as shown in Fig. 2b . We remark on two aspects of these curves: (i) although these SRO samples are much less active, the OER is still structure sensitive, with SRO(111) showing greater activity than SRO(001); and (ii) the structure sensitivity is more pronounced for the samples with low conductance. Based on the results in Fig. 2a,b , we conclude that surface chemistry is not affected by the difference in conductance; the latter controls only the dynamics and the potential window of changes in surface morphology and electronic properties, as discussed further below. The changes in surface morphology were established by monitoring variations in the specular rod at electrode potentials held to values just below and above the OER. In Fig. 2c–e , we present results for a (low conductance) SRO(001) film that illustrate the evolution of the film structure as a function of potential. (Recall, that in order to avoid variations arising from the ‘synthesis technique’ for high-conductance samples, we have used the unmodified low-conductance films for all the discussions in the manuscript. The impact of the conductivity of the samples is discussed in detail in the Methods section and Supplementary Fig. 3 .) Results for the SRO (111) film follow the same trend, as summarized in Supplementary Fig. 4 . The X-ray scattering data in Fig. 2d reveal clearly observable KF for potentials between 0.95 and 1.1 V, indicating that within this electrode potential window, the smooth and atomically flat SRO(001) film is stable. Above 1.1 V, however, the fringe contrast decreases and nearly disappears by 1.45 V, signaling considerable roughening of the surface [36] . This was confirmed from an ex situ AFM image acquired after exposing the electrode to 1.45 V ( Supplementary Fig. 5 ); the roughened surface exhibits many nano-sized islands randomly distributed on the surface. Another notable feature in Fig. 2d is that even after 30 min at 1.45 V, the SRO(001) film peak was still clearly visible in a specular rod scan, implying that the film was not completely dissolved under these conditions. However, from Fig. 2d (see the green dashed line), it is also evident that after an extended hold at 1.45 V, the SRO(001) film will completely degrade, suggesting that dissolution/roughening of low-conductance oxide is mainly controlled by the high resistance. Further analysis, summarized in Fig. 2e , reveals that while a dissolution rate of ~2.5 unit cells h −1 is observed for SRO(001) films, the dissolution rate of the SRO(111) is much faster (~15.6 unit cells h −1 at 1.35 V). The difference in the dissolution rate between these two orientations can be understood largely in terms of a difference in the electronic and morphological properties of SRO films, as discussed below. Insight into the impact of potential-induced structural degradation (roughening and/or dissolution) on electronic properties (that is, the change in the oxidation state of Ru cations) can be obtained from a series of measurements performed with X-ray absorption near-edge spectroscopy (XANES) [43] . For SRO(001), the XANES spectrum at 0.95 V is consistent with the Ru 4+ oxidation state, as expected for stoichiometric SrRuO 3 ( Fig. 2c ). The data also show that up to a potential of 1.4 V, there is no measurable change in the Ru valence state, as determined by the lack of a shift in the position of the Ru K-edge. The fact that the film roughness and structure remain unchanged in this potential region ( Fig. 2d ) implies that the Ru +4 state is stable up to 1.4 V. Above this potential, however, there is a drastic change in the Ru K-edge line shape as well as the emergence of a weak, but clearly visible pre-peak (inset of Fig. 2c ). These variations are consistent with a change in the Ru valence state (denoted as n hereafter) from oxidation state of n =4 to a value of n >4+ (Ru n>4+ ) ( Supplementary Fig. 6 ). Although it is not possible to unambiguously determine the exact value of the Ru oxidation state at the surface of the films, we can determine the average oxidation state of Ru cations in the bulk of the films (which is not potential dependent and is in the n =4+ state) as well as in the (near)surface region that we assign as Ru n>4+ . An intriguing aspect of the results shown in Fig. 2 concerns a possible correlation between surface morphology and the potential-induced variation of the Ru oxidation state. A comparison between Fig. 2c,d sheds light on such a correlation for the SRO(001) film; namely, the observed decrease in structural integrity (stability) is concomitant with the valence state transformation from Ru 4+ to Ru n>4+ . Additional in situ studies of the (110) and (111) orientations show that they follow the same trends as the (001) film, differing only in the kinetics of the dissolution process ( Supplementary Fig. 4 ) and the onset potential at which this transition is observed. For example, a close inspection of Fig. 2a,c reveals that an ‘ordered(Ru 4+ )-to-disordered(Ru n>4+ )’ transition is strongly structure sensitive with the onset potential increasing from more defective films with the (111) orientations to highly ordered and less defective (001) film. Based on the above results, we conclude that while the Ru 4+ state appears to be stable in all three SRO(hkl) structures, the Ru n>4+ state is unstable leading to dissolution of Ru. The rate of this transition is influenced by surface defects either being inherently present on the as-grown films (structural effects) or even created by the potential-induced adsorption of oxygenated surfaces (electronic effects). The question naturally arises as to how the ‘ordered(Ru 4+ )-to-disordered(Ru n>4+ )’ transition may affect the OER. The OER in alkaline environments (4OH − =O 2 +2H 2 O+4e − ) is a rather complex process, involving the formation of many reaction intermediates before OH − is completely transformed to O 2 and H 2 O [2] , [25] , [44] , [45] , [46] . From experiments on high-surface area perovskites, it was established that in alkaline solutions the activities correlate well with the occupancy of 3d surface orbitals with e g symmetry [25] . In contrast to the catalytic concerns, however, relatively little fundamental understanding exists regarding the degradation mechanism of oxide anode materials during the OER [14] , [47] , [48] , [49] , as well as how these morphological changes may affect the rate of the OER. In the following, we demonstrate that understanding the coupling between the dissolution of SRO(hkl) thin films and catalytic properties is essential to taking the next critical step—the selection of new materials that one would exhibit both optimal reactivity and stability. Therefore, beyond the question of reactivity of the SRO(hkl) films for the OER, a central issue of this work concerns stability–activity relationships that have been rarely discussed (at least not at atomic levels) in electrocatalysis on oxide surfaces, a notable exception being the recent work of Grimaud et al. [50] on the double perovskites. Therefore, by exploring variations in the oxidation state of Ru active centres, the triggered dissolution of Ru cations via the electrode potential (resulting in formation of defect sites), and the concomitant evolution of O 2 on SRO(hkl) surfaces, much can be learned regarding a functional link between the oxidation state of active centres, their stability and their reactivity that is utterly inaccessible when studying high-surface area oxide materials. Structure–function relationships Probing SRO samples with low conductance offers several virtues, in particular slowing the dissolution of active Ru components and hence allowing the role of film structure on stability/activity to be obtained in a more direct fashion simply by comparing the activity for the OER ( Fig. 3a ), the stability of the films via inductively coupled plasma-mass spectroscopy (ICP) measurements ( Fig. 3e ), the change in valence by X-ray spectroscopy ( Fig. 2c and Supplementary Fig. 6 ), and the variations in structural properties (for example, roughening of the film) during the OER ( Fig. 3b–d ). From Fig. 3a , it is evident that the activity increases in the order (001)<(110)<(111); this is inversely related to the observed stability of the Ru and Sr cations ( Fig. 3e ). Interestingly, the shape of polarization curves in Fig. 3a is markedly different from the one presented in Fig. 2a for SRO samples with low conductance. For all three SRO(hkl) films in Fig. 3a , an initial logarithmic increase in current density (typically observed for the OER) is followed first by currents that appear to be ‘diffusion-limited’ and then by a fast deactivation (which was also observed on samples with high conductivity). Note that the deactivation is also highly structure sensitive [(001)<(110)<(111)]. Given that no measurable activity is observed during the second potential sweep ( Fig. 2a ), Ru appears to completely dissolve from the film during the first sweep. This, in turn, suggests that the unusual shape of the polarization curves in Fig. 3a is governed by an intimate relationship between the formation of unstable Ru n>4+ sites (see above), the structure-dependent dissolution of Ru n>4+ and the concomitant evolution of O 2 on the active sites that are created upon Ru n>4+ dissolution. The complete loss in OER activity after a single potential sweep also suggests that during the OER, there is no redeposition of Ru onto the SRO electrode, an important observation that will be further documented below. 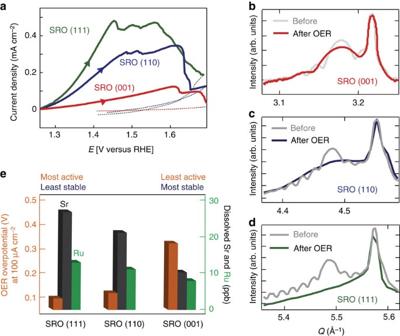Figure 3: Structure–functional relation of SRO films for the oxygen evolution reaction (OER). (a) Decreases of current density measured at certain potentials: 1.44, 1.48 and 1.61 V for SRO(111), (110) and (001), respectively. (b–d) Structural changes of SRO films after the OER measurements: (b) more than 30% decrease of the thickness of the SRO(001); (c) 60% for the SRO(110); and (d) 90% for the SRO(111) film. (e) Structural dependence of activity and stability (dissolved Sr (black) and Ru (green) amount) in SRO films, measured by OER overpotential (red) at 100 μA cm−2and ICP measurement. Activity: SRO(111)>SRO(110)>SRO(001); stability: SRO(001)>SRO(110)>SRO(111). Figure 3: Structure–functional relation of SRO films for the oxygen evolution reaction (OER). ( a ) Decreases of current density measured at certain potentials: 1.44, 1.48 and 1.61 V for SRO(111), (110) and (001), respectively. ( b – d ) Structural changes of SRO films after the OER measurements: ( b ) more than 30% decrease of the thickness of the SRO(001); ( c ) 60% for the SRO(110); and ( d ) 90% for the SRO(111) film. ( e ) Structural dependence of activity and stability (dissolved Sr (black) and Ru (green) amount) in SRO films, measured by OER overpotential (red) at 100 μA cm −2 and ICP measurement. Activity: SRO(111)>SRO(110)>SRO(001); stability: SRO(001)>SRO(110)>SRO(111). Full size image In general, it is very difficult to unambiguously distinguish between many different processes occurring during particular reaction, a typical example being metal deposition always accompanied by the simultaneous desorption of specific, adsorbed anions [51] , [52] . In the case of the OER, there are published rotating ring disk electrode (RRDE) results [53] that indicated that the OER on Ru always go together with Ru dissolution. In order to provide further insight into relationships between the OER and the concomitant dissolution of Ru, we apply the very same RRDE method to probe the stability of Ru and the OER activity (more details on the RRDE and X-ray photoemission spectroscopy results can be found in the Supplementary Note 1 and Supplementary Figs 7 and 8 ). Owing to technical limitations in the assembly of the RRDE apparatus with SRO samples in the disk position, we instead performed experiments with a Ru bulk electrode in the disk configuration and a ruthenized platinum ring used to ‘collect’ the dissolved Ru cations. However, the findings with a pure Ru electrode can, at least qualitatively, be used to understand the processes at the SRO(hkl) thin film electrodes. Two distinctive features in Supplementary Fig. 7 are noteworthy: (i) the OER is always accompanied by Ru dissolution; and (ii) the anodic current measured on the disk electrode is two orders of magnitude higher than the corresponding corrosion current measured on the ring electrode, implying that contribution of a current corresponding to Ru dissolution to the OER is ~10%. We thus conclude that the measured anodic currents on the disk electrode are mainly (90%) owing to the OER. Returning to SRO(hkl) systems, we suggest that key conclusions obtained from the RRDE in Supplementary Fig. 7 are applicable to all three SRO films, at least qualitatively. This contention is supported by the fact that changes in the oxidation state of Ru measured by X-ray photoemission spectroscopy [14] are identical with those established for the SRO(hkl) thin films. Therefore, we propose that, as for the Ru bulk electrode, the measured anodic currents are mainly due to the OER and not the dissolution of Ru. Another fundamental question concerns structural changes after the OER on SRO(hkl) films. Ex situ specular rod measurements acquired before and after a potential excursion up to 1.75 V are shown in Fig. 3b–d . Again, changes in film morphology are strongly structure sensitive. For example, the retention of both KF and a film peak for the SRO(001) sample after the OER ( Fig. 3b ) is a clear indication that although the surface is roughened, the film remains a single crystal. Figure 3c shows that for the SRO(110), only a very broad film peak is observed after the OER, indicating that the film is much thinner and very rough, and thus less stable than the (001). Since no Bragg peak appears for the SRO(111) film after the OER ( Fig. 3d ), we conclude that (111) films are very unstable after exposure to potentials above 1.45 V. As discussed further below, these behavioural differences support directly that SRO films are very unstable in the potential region where the OER occurs. The correlation between the activity of the OER (expressed as a measured overpotential at a constant current density, 100 μA cm −2 ) and stability (evaluated by quantifying the dissolution of Sr and Ru cations) for the SRO(hkl) films is summarized in Fig. 3e . The fact that the very same activity–stability trends are observed on high-conductance samples ( Supplementary Fig. 9 ), it justifies our decision to focus more on the SRO systems with lower conductance but higher stability. Clearly, the activity of the OER increases in the order (001)<<(110)<(111), demonstrating an important structural effect. Figure 3e also shows that (i) for all SRO(hkl) systems, the solution concentration of Sr is always higher than that of Ru, implying that the dissolution rates are different or due to limitations of the ICP measurements; and (ii) the stability of the SRO films increases in the order (111)<(110)<<(001). Hence, there is a strong inverse correlation between activity and stability, a relationship that has not, to our knowledge, been considered in the analysis of the OER on any oxide surface. On what basis, then, can we rationalize the inverse relationship observed for stability and activity in Fig. 3e ? To begin to unravel the rich complexity of the relationships between the activity of the OER and the concomitant stability of SRO(hkl) surfaces, we point out that several studies have unambiguously shown that the stability of oxide surfaces is closely related to both the density of surface defects [54] as well as the energy and polarity of the oxide planes [55] . Since it is very difficult to decouple morphological and electronic effects in (electro)catalysis, it would be very difficult to unambiguously determine which of these two properties may govern the observed structure–function relationships. The importance of surface defects is well documented for metal–electrolyte interfaces [56] , [57] ; for example, many anomalous activities observed on single-crystal metal surfaces in electrochemical systems were found to be predominately governed by characteristic types of surface defects. The same applies to the noble metal oxides, for example, crystalline thermal oxides are always much less active than highly defective electrochemically made oxides [54] . Based on the fact that SRO(001) is the least defective surface, it is also plausible that the (001) surface is the least active simply because it contained the least number of defect sites. Besides a morphological effect, the stability/activity of SRO films may also be controlled by the Sr-oxide and Ru-oxide polarity. In the ionic limit, while (001)-oriented SRO films are non-polar, the (110)- and (111)-oriented films are both polar as they are formed from alternating (SrRuO) 4+ /(O 2 ) 4− and (SrO 3 ) 4+ /(Ru) 4− planes, respectively. Given that any residual polarity would increase the surface energy, surfaces such as the SRO(110) and SRO(111) should be more unstable than the corresponding non-polar (001). In brief, using the bond valence method ( Supplementary Note 2 ) for assessing the relative strengths of the Sr–O and Ru–O bonds, it can be determined that the surface energy of SRO increases in the order (001) « (110)<(111), with the energies of the (110) and (111) considerably larger than that for (001) [58] (more information is provided in the Supplementary Notes 2 and 3 ). We note that under-coordinated polar surfaces such as the (110) and the (111) provide additional adsorption sites (in our case for the adsorption of OH − ) and are typically more reactive [59] . The subject of chemical anisotropy at oxide surfaces has been explored for some time with photocatalytic reactions [60] , and very recently for oxygen surface exchange [61] . In the latter studies, the (001) perovskite surface always exhibited the slowest exchange rates because of its relatively high stability. However, in all of these studies, there was very little microscopic understanding of the relationship. Based on the above results and discussion, we propose that both Sr and Ru are more stable for the highly ordered (morphological effect) and low-energy (electronic effect) SRO(001) surfaces than for the more defective, high-energy surfaces with the (110) and (111) orientations. The degradation of the SRO films may be controlled by a combination of the electrochemical dissolution of Ru and the chemical corrosion of Sr [62] . Although the physical origin and behavioural details of the degradation of SRO(hkl) are difficult to assess (studies along these lines are highly hypothetical even for ‘simple’ monometallic oxides such as Pt and/or Ru oxides), in the following, we explore the manner and extent to which the applied potential may influence the dissolution of Sr and Ru. Our analysis will be based on four experimental facts. First, while the Ru 4+ state appears to be stable in all three SRO(hkl) structures, the Ru n>4+ state is unstable leading to the dissolution of Ru ( Figs 2 and 3 ). Second, the OER is always accompanied with the Ru dissolution, supported by our RRDE studies with bulk Ru electrode. Third, the contribution of the Ru dissolution current to the total is rather small; according to RRDE analyses, ~90% of the measured current is due to the OER. Fourth, in contrast to SRO, we found that both Sr and Ti are highly stable in Nb-doped STO films ( Supplementary Table 1 ); not surprisingly, we also found that the STO(hkl) surfaces are highly inactive for the OER. Our experiments with STO unambiguously show that Sr is stable if the B-site in the perovskite structure (Ti) is stable; however, if the B-sites are unstable, as in the case of Ru n>+4 in SRO, then Sr also becomes highly unstable and dissolves into the electrolyte. Although it is not clear at this moment why the chemical dissolution of Sr is higher than Ru, we do have wealth of electrochemical, analytical, spectroscopic and structural information that help to establish, at atomic levels, relationships between the potential control variations in the Ru oxidation state and the nature of the Ru cations in determining the stability of SRO(hkl) surfaces that, in turn, is governing the kinetics of the OER. Overall, then, the SRO single-crystal films studied in this work offer a unique opportunity to discover the functional links between stability and reactivity on SRO(hkl) films in electrochemical environments. Our results show that the degradation of SRO films coincides with the electrode potential at which Ru n>4+ is observed, so we suggest that irrespective of the surface orientation the Ru n>4+ is the ‘active centre’ that is unstable in electrochemical environments. The dissolution of Ru is governed by a combination of morphological (surface density of defects) and electronic (surface energy) effects, which are difficult to decouple. As a consequence, the stability of SRO films increases from high energy, more defective films with the (110) and (111) orientations to the highly ordered, low-energy (001) film. We also show that the OER on SRO(hkl) is always accompanied by dissolution of the corresponding cations, so that in addition to the pure ‘energetic factors’, the selection of these types of materials for the OER must strike a balance between two opposing effects—the balance between active but unstable sites with stable and inactive sites. The fact that the order in activity is inverse to the order in stability, suggests that the OER on SRO(hkl) is controlled by the surface density of defects (for example, stability of Ru cations) rather than the binding energy between the substrate and the reactants, intermediates and products. We conclude that detailed studies necessary to unravel relationships between stability and activity of oxide surfaces in electrochemical environments can be helpful in the design of new oxide materials that can be active and stable in both aqueous environments and organic solutions. Thin film synthesis Epitaxial SrRuO 3 (SRO) films were prepared by radio-frequency magnetron sputter deposition (AJA International, Inc.) onto 0.5 wt.% Nb-doped SrTiO 3 (Nb:STO) single-crystal substrates (6 mm diameter and 0.5 mm thick; CrysTec GmbH) with three orientations: (001), (110) and (111). Before deposition, the Nb:STO substrates were etched using buffered HF and annealed at 950 °C for 3 h in flowing oxygen to control the termination of the substrates [63] . The SRO films were deposited at 650–750 °C and 15 mTorr oxygen partial pressure. The As-deposited films were post-annealed in the sputtering chamber at 50–100 mTorr. The quality of the films was verified by X-ray absorption spectroscopy (Ru 4+ ) and electrical measurements (ferromagnetic behaviour below 150 K) at Sectors 12BM and 12ID-D, the Advanced Photon Source (APS) and Center for Nanoscale Materials, Argonne National Laboratory. For the in situ X-ray scattering and spectroscopy measurements at APS, several epitaxial SRO films were characterized with thicknesses ranging from 10 to 30 nm, all of which remained coherently strained with the substrate. Electrochemical characterization Electrochemical measurements were performed using an Autolab PGSTAT 302N potentiostat. The thin film composite electrode was lightly pressed into a custom-made removable rotating disc electrode collet that isolated and held the SRO surface to the electrolyte and allowed electrical contact to the back of the sample with a stainless steel spring. The rotating disc electrode collet containing the sample was rinsed and transferred to a standard three-compartment electrochemical cell containing Ar-saturated 0.1 M KOH (Sigma-Aldrich). During the experiments, the electrode was either immersed under potential control at 0.05 V (for cyclic voltammetry and some in situ X-ray electrochemical measurements) or 0.8 V (typical open circuit voltage, for OER and some in situ X-ray electrochemical measurements). All activity measurements were iR compensated for the solution resistance at 1,600 r.p.m., using a 5-mV s −1 scan rate in a potentiodynamic positive-going sweep. The iR compensation removed resistance from the solution and other constant resistances (typically ~38 Ω), not from the sample. We also performed chronopotentiometric experiments in which we found that the OER activities dropped rapidly because of fast dissolution of Ru and Sr cations, making it difficult to obtain accurate measures, so we decided to present only potendiodynamic results. An Ag/AgCl reference electrode was used in all experiments; all reference potentials in this paper were corrected to the reversible hydrogen electrode scale. A gold counter electrode was used to minimize contamination from more active materials on the working electrode surface, but it is still possible that Ru deposits onto the counter electrode and the cell wells during Ru dissolution. Note that the apparent ‘diffusion-limited’ currents for the OER, in Figs 2a and 3a , arise from dissolution currents overcoming the OER current as active sites are lost. Electrical contact For the electrochemical measurements and epitaxial film growth, we used 0.5 wt.% Nb-doped STO single-crystal substrates that are a highly conducting oxide substrate at room temperature. The conductivity of Nb:STO is ~50 Ω −1 cm −1 at room temperature (CrysTec GmbH), comparable with that of glassy carbon. In order to form an ohmic contact between the Nb:STO and a working electrode, Ti and Pt were deposited on the back of the substrate by sputter deposition. The interface between SRO (work function: 5.2 eV) and Nb:STO (n-type semiconducting behaviour) forms a Schottky junction, showing rectifying behaviour [64] . This Schottky barrier can make the Nb:STO/SRO sample highly resistant (>1 kΩ—100 MΩ, measured at 0.1 V). To modify the conductance of the samples, we prepared two types of Nb:STO/SRO samples: (1) SRO films having a SC between the SRO top surface and the backside of the substrate by metal deposition onto the side wall (SRO(hkl)|SC); and (2) SRO films without the SC (SRO(hkl)). The effective resistance of SRO(hkl) is 5–10 times higher than that of SRO(hkl)|SC owing to the existence of the Schottky barrier ( Supplementary Fig. 3 ). Ex situ and in situ X-ray electrochemical study X-ray measurements were performed using a Huber six-circle diffractometer at Sector 12ID-D of the APS. For X-ray reflectivity and diffraction measurements, both point (Cyberstar) and 2D (PILATUS, Dectris) detectors were used. Ru K-edge XANES measurements were performed with a VORTEX silicon drift detector (SII) in fluorescence mode. The in situ X-ray electrochemical cell was designed for use with 6 mm diameter, 0.5-mm-thick single-crystal substrates with a Ag/AgCl reference electrode. The sample sits in a Kel-F collet that holds the sample while allowing a back contact to be made with Pt wire. More than 10 in situ samples have been studied to check the reproducibility, over a 2-year span at APS. We also performed ex situ X-ray diffraction using a lab source diffractometer (Bruker D8 Advance) with monochromatized Cu-K α radiation ( λ =1.54 Å). The data shown in Fig. 2e were extracted from fits to the specular rod data shown in Fig. 2d , using a fitting procedure based on simple structural models [65] ( Supplementary Fig. 10 ). Inductively coupled plasma–mass spectrometry For the inductively coupled plasma–mass spectrometry (ICP; PerkinElmer/SCIEX ELAN DRC-II) measurements, we sampled the electrolyte at the end of the positive-going potentiodynamic OER scan by withdrawing the electrode to prevent redeposition of the dissolved products. How to cite this article: Chang, S. H. et al. Functional links between stability and reactivity of strontium ruthenate single crystals during oxygen evolution. Nat. Commun. 5:4191 doi: 10.1038/ncomms5191 (2014).